An intrinsically labile α-helix abutting the BCL9-binding site of β-catenin is required for its inhibition by carnosic acid Wnt/β-catenin signalling controls development and tissue homeostasis. Moreover, activated β-catenin can be oncogenic and, notably, drives colorectal cancer. Inhibiting oncogenic β-catenin has proven a formidable challenge. Here we design a screen for small-molecule inhibitors of β-catenin's binding to its cofactor BCL9, and discover five related natural compounds, including carnosic acid from rosemary, which attenuates transcriptional β-catenin outputs in colorectal cancer cells. Evidence from NMR and analytical ultracentrifugation demonstrates that the carnosic acid response requires an intrinsically labile α-helix (H1) amino-terminally abutting the BCL9-binding site in β-catenin. Similarly, in colorectal cancer cells with hyperactive β-catenin signalling, carnosic acid targets predominantly the transcriptionally active ('oncogenic') form of β-catenin for proteasomal degradation in an H1-dependent manner. Hence, H1 is an 'Achilles' Heel' of β-catenin, which can be exploited for destabilization of oncogenic β-catenin by small molecules, providing proof-of-principle for a new strategy for developing direct inhibitors of oncogenic β-catenin. Wnt signalling induces a context-specific transcriptional programme, which controls numerous developmental processes and adult stem cell niches [1] . In the absence of Wnt, the key effector of this pathway, β-catenin, is continuously degraded. Axin together with the Adenomatous polyposis coli (APC) tumour suppressor promotes the phosphorylation of β-catenin by glycogen synthase kinase 3 (GSK3), which earmarks it for proteasomal degradation. If this fails in the colonic epithelium, because of inactivating mutations of APC , β-catenin is stabilized inappropriately and thus initiates tumourigenesis. Moreover, mutations in the phosphorylation sites of β-catenin have been found in many other cancers [2] . Unphosphorylated β-catenin accumulates and associates with the DNA-binding T-cell factor/lymphoid enhancer factors (TCF/LEF), to recruit a range of transcriptional co-activators to its carboxy terminus [3] . The transcriptional switches induced by β-catenin-TCF are the key outputs of Wnt/β-catenin signalling, and determine both normal and malignant cell fates [1] . Below, we use 'activated' or 'oncogenic' interchangeably, referring to unphosphorylated transcriptionally active β-catenin. The case for β-catenin as a target for therapeutic intervention in cancer is overwhelming. However, developing direct inhibitors of oncogenic β-catenin has proven a formidable challenge: there are no well-established enzymatic activators of β-catenin that could be inhibited, and its main ligand interaction surface is extensive and shared between positive and negative regulators [4] . Nevertheless, there have been several successes in developing indirect small-molecule inhibitors of oncogenic β-catenin, which reduce its activity or stability by targeting one of its regulators [5] , [6] , [7] , [8] . BCL9 proteins and their molecular interfaces with β-catenin and Pygo proteins have emerged as promising new targets for interference in cancer. BCL9 proteins are adaptors between β-catenin and Pygo [9] , and assist their Pygo cofactors in recognizing modified histone H3 tails by their plant homeodomain (PHD) fingers [10] . BCL9 and Pygo thus promote β-catenin-mediated transcription during normal development and in colorectal cancer cells [9] , [11] , [12] , [13] , [14] . BCL9 can be overexpressed in cancers and exhibits tumour-promoting effects in mouse xenograft models [15] . Mouse knockout studies have uncovered key roles of Bcl9 and Pygo2 in controlling β-catenin-dependent transcription of stem cell markers in normal intestinal crypts and neoplasias [16] , and in the mammary progenitor cell compartment [17] . Indeed, Pygo is one of the targets destabilized by a small-molecule kinase agonist [6] . Here we focus on BCL9 and its interaction with β-catenin. We developed an ELISA-based 'plus–minus' assay to screen for small compounds that disrupt selectively the binding of β-catenin to BCL9 without affecting its binding to TCF. We thus identified a small group of chemically related natural compounds, one of which, carnosic acid (CA) from rosemary, acts in a dose-dependent manner to inhibit BCL9-β-catenin binding in vitro , and β-catenin-dependent transcription in colorectal cancer cells. Our biophysical analysis pinpointed a key element required for the CA response, namely a structurally labile α-helix (H1) at the amino terminus of the β-catenin Armadillo repeat domain (ARD), abutting the BCL9-binding site. We provide evidence that CA acts through H1 to exacerbate an intrinsic tendency of the ARD N-terminus to aggregate, thus attenuating in vitro binding to BCL9. In vivo , CA promotes selectively the proteasomal degradation of unphosphorylated β-catenin in an H1-dependent manner. H1 is thus an Achilles' Heel of β-catenin, and our discovery of a β-catenin-destabilizing compound provides proof-of-principle for new strategies to identify direct small-molecule inhibitors of oncogenic β-catenin. A screen for inhibitors of the β-catenin-BCL9 interaction The BCL9 homology domain 2 (HD2) binds to the first repeat of the ARD [9] , [18] , which is critical for β-catenin-dependent transcription in colorectal cancer cells [14] . To identify inhibitors of this interaction, we developed an in vitro assay that monitors the binding of His-HD2 to glutathione S-transferase (GST)-ARD (immobilized on glutathione-coated microplates), using a colorimetric assay to quantify bound His-HD2 after addition of compounds ( Fig. 1a ). Competition with untagged soluble ARD or HD2 shows dose-dependent saturable inhibition, whereas chymotrypsin has no effect ( Fig. 1b ). L363F and L366K HD2 mutants (defective in β-catenin binding [14] ) show reduced binding to GST-ARD ( Fig. 1c ). Importantly, we also monitored the binding of the N-terminus of TCF-4 (His-nTCF) to GST-ARD ( Fig. 1a ), as a 'counter-screen' to remove unspecific hits. 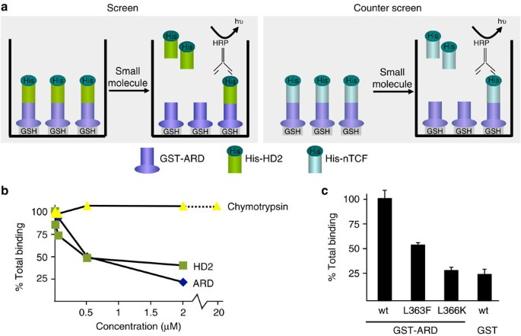Figure 1: A plus–minus screen for compounds blocking ARD-HD2 binding. (a) Schematic illustration of the assay format. Screen: GST-ARD was bound to glutathione-coated plates, to which His-HD2 is added, to allow complex formation. On incubation with compounds, and subsequent washes, bound His-HD2 was detected with horse radish peroxidase (HRP)-coupled α-His andO-phenylenediamine (Phytopure and LOPAC screens), or POD substrate (MRCT screen; seeSupplementary Fig. S2). Counter-screen: His-nTCF was used instead of His-HD2. (b) Dose-dependent inhibition of binding between plate-bound GST-ARD and His-HD2 with increasing concentrations of soluble ARD or HD2; binding was not affected by 0.5–20 μM chymotrypsin. (c) Binding of wild-type (wt) and mutant His-HD2 to GST-ARD, or to GST, as indicated; error bars, standard deviations (n=4). Figure 1: A plus–minus screen for compounds blocking ARD-HD2 binding. ( a ) Schematic illustration of the assay format. Screen: GST-ARD was bound to glutathione-coated plates, to which His-HD2 is added, to allow complex formation. On incubation with compounds, and subsequent washes, bound His-HD2 was detected with horse radish peroxidase (HRP)-coupled α-His and O -phenylenediamine (Phytopure and LOPAC screens), or POD substrate (MRCT screen; see Supplementary Fig. S2 ). Counter-screen: His-nTCF was used instead of His-HD2. ( b ) Dose-dependent inhibition of binding between plate-bound GST-ARD and His-HD2 with increasing concentrations of soluble ARD or HD2; binding was not affected by 0.5–20 μM chymotrypsin. ( c ) Binding of wild-type (wt) and mutant His-HD2 to GST-ARD, or to GST, as indicated; error bars, standard deviations ( n =4). Full size image We thus screened two 1250-compound libraries—LOPAC (known pharmacological inhibitors) and Phytopure (chemically diverse natural compounds), obtaining similar Z ′ values and hit rates for the primary screens ( Supplementary Table S1 ). All LOPAC hits also scored positive in the counter-screen, and were thus discarded as non-selective. However, three phytopure hits with similar K i values for HD2-ARD binding ( Supplementary Fig. S1 and Table S2 ) did not score in the counter-screen. Two of these harbour a common catechol core, allowing us to identify three related compounds in the PubChem database ( Fig. 2a ): totarol, CA and carnosol (CO). Totarol nonspecifically precipitated the proteins in our assay, and was therefore discarded. CA and CO inhibited HD2-ARD binding dose dependently ( Fig. 2b ), with K i values of 3.3±1.8 μM and 8.2±4.3 μM, respectively ( Supplementary Table S2 ), but only CA was specific. CO also inhibited nTCF-ARD binding ( K i 23±15 μM; Supplementary Table S2 ) and so did not pass this specificity test. 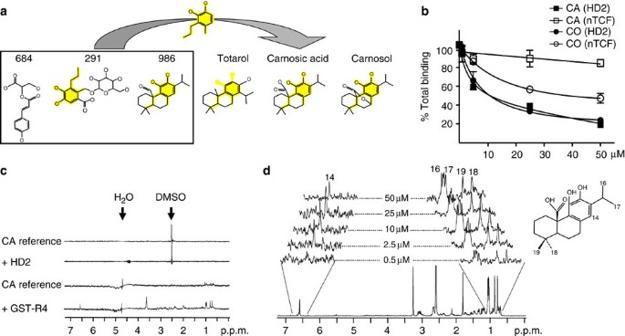Figure 2: CA inhibits the BCL9-β-catenin interaction. (a) Structure of Phytopure hits (986, 291, 684) and chemical relatives; catechol cores are in yellow. (b) Dose-dependent inhibition of HD2-ARD binding by CA and carnosol (CO); error bars, standard deviations (n=4). (c,d) STD spectra of CA references (50 μM), (c) matched to CA+10 μM GST-R4 or HD2, or (d) 0.05–50 μM of GST-R4, as indicated (see alsoFig. 4b); the1H spectrum of CA is shown underneath. Figure 2: CA inhibits the BCL9-β-catenin interaction. ( a ) Structure of Phytopure hits (986, 291, 684) and chemical relatives; catechol cores are in yellow. ( b ) Dose-dependent inhibition of HD2-ARD binding by CA and carnosol (CO); error bars, standard deviations ( n =4). ( c , d ) STD spectra of CA references (50 μM), ( c ) matched to CA+10 μM GST-R4 or HD2, or ( d ) 0.05–50 μM of GST-R4, as indicated (see also Fig. 4b ); the 1 H spectrum of CA is shown underneath. Full size image We adapted this format for higher throughput, to screen the 45,000-compound MRC Technology (MRCT) library, by switching to a 384-well format and changing the detection method to luminescence-based, which produced a more robust assay ( Z ′=0.70; Supplementary Fig. S2 ). This identified 12 hits, each of which scored positive in the counter-screen and so were discarded ( Supplementary Table S1 ). We thus focussed on CA for subsequent analysis. CA binds to the ARD N-terminus To identify the target of CA, we used NMR saturation transfer difference (STD) spectroscopy as a highly sensitive method to probe the interaction between CA and its target domain. As the ARD is large, we decided to use the minimal HD2-binding domain within its N-terminus [9] , that is, its first four repeats (called R4): R4 binds to HD2 with similar affinity as ARD [18] ( Supplementary Table S3) , and the K i values for CA-mediated inhibition of GST-R4-HD2 and GST-ARD-HD2 are identical. We next sought to confirm that R4 forms a well-structured ARD subdomain, and thus solved its crystal structure in its apo form, and in complex with HD2, at 2.5 and 2.2 Å resolution, respectively ( Supplementary Table S4 ). These structures superimpose very well on each other, and onto the corresponding segments of the ternary ARD-HD2–nTCF complex [18] and of the ARD itself [19] , with root-mean-square deviation values of 0.41–0.54 Å ( Supplementary Table S4 ). Notably, the first α-helix (H1) of the ARD is unstructured in the crystal, but H1 adopts a helical structure when in complex with HD2 ( Supplementary Fig. S3 ), as previously observed [18] . The high similarities between these structures further validated our use of R4 for functional analysis. To identify the CA-binding domain, we performed STD assays with purified R4 or HD2 +/− CA. R4 tested positive in this ligand-observed binding assay whereas HD2 was negative ( Fig. 2c ). Titration with varying concentrations of R4 ( Fig. 2d ) indicates saturable binding ( Supplementary Fig. S4 ), allowing us to estimate a K d in the low micromolar range (5–20 μM). Importantly, these STD assays unequivocally identify R4 as the molecular target of CA. CA exacerbates an intrinsic tendency of R4 to aggregate To further characterize the interaction between CA and R4, we acquired 1 H– 15 N heteronuclear single-quantum correlation (HSQC) spectra. 15 N-Labelled HD2 produces well-resolved H N –N correlation peaks corresponding to its 49 non-proline backbone amides ( Supplementary Fig. S5 ), with homogeneous peak intensities across the spectrum ( Fig. 3a ), consistent with a well-folded helical domain [18] ( Supplementary Fig. S3 ). This spectrum is unchanged by stoichiometric (that is, >10 times K i ; Supplementary Table S2 ) addition of CA ( Fig. 3a ; Supplementary Fig. S5 ), confirming that CA does not bind to HD2. 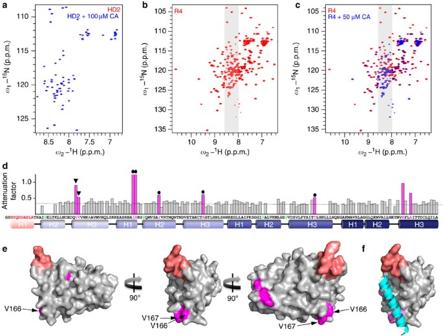Figure 3: R4 contains the molecular target of CA. (a) Overlay of HSQC of15N-labelled HD2+CA (100 μM each) onto15N-labelled HD2 (100 μM) with solvent only, as indicated. (b) HSQC of15N-labelled R4 (50 μM); (c) overlay of15N-labelled R4+CA (50 μM each) onto15N-labelled R4 (50 μM) with solvent only, as indicated; the 8.0–8.6 p.p.m. range of proton chemical shifts is shaded in grey. (d) Map of CA-induced attenuation factors derived fromconto individual R4 residues (α-helices, cylinders underneath sequence; red, H1 residues; green, prolines); attenuation factors were calculated from peak signal intensities of R4/R4+CA (purple, attenuation of signal intensity >2 standard deviations above average of CA-induced reduction of overall signal intensity, indicated by dashed line); 123/138 peaks from the assigned R4ΔH1spectrum (Supplementary Fig. S6) were scored (black dots, N-terminal R4 core residues; arrows, HD2-binding surface residues). (e,f) Projections of CA-induced intensity changes, colour-coded as inc, onto the R4 apo structure (f, with HD2 added; see alsoSupplementary Fig. S3); valines at the HD2-binding site are labelled. Figure 3: R4 contains the molecular target of CA. ( a ) Overlay of HSQC of 15 N-labelled HD2+CA (100 μM each) onto 15 N-labelled HD2 (100 μM) with solvent only, as indicated. ( b ) HSQC of 15 N-labelled R4 (50 μM); ( c ) overlay of 15 N-labelled R4+CA (50 μM each) onto 15 N-labelled R4 (50 μM) with solvent only, as indicated; the 8.0–8.6 p.p.m. range of proton chemical shifts is shaded in grey. ( d ) Map of CA-induced attenuation factors derived from c onto individual R4 residues (α-helices, cylinders underneath sequence; red, H1 residues; green, prolines); attenuation factors were calculated from peak signal intensities of R4/R4+CA (purple, attenuation of signal intensity >2 standard deviations above average of CA-induced reduction of overall signal intensity, indicated by dashed line); 123/138 peaks from the assigned R4 ΔH1 spectrum ( Supplementary Fig. S6 ) were scored (black dots, N-terminal R4 core residues; arrows, HD2-binding surface residues). ( e , f ) Projections of CA-induced intensity changes, colour-coded as in c , onto the R4 apo structure ( f , with HD2 added; see also Supplementary Fig. S3 ); valines at the HD2-binding site are labelled. Full size image The HSQC of 15 N-labelled R4 is well dispersed, exhibiting >130 resolvable peaks ( Fig. 3b ). However, in contrast to HD2, we observe unequal peak intensities across the R4 spectrum: peaks within the 8–8.6 p.p.m. range of the 1 H axis ( Fig. 3b , shaded grey) tend to be stronger, broader and poorly resolved, compared with those outside this range, indicative of aggregation. Indeed, NMR relaxation properties of R4 ( 1 H T 2 relaxation time constants, as measured from one-dimensional spin-echo [20] ) are consistent with a molecular mass of >65 kDa (expected monomer mass 21 kDa), supporting the notion of R4 oligomerization, although we emphasize that R4 remains predominantly monomeric at the concentrations used for NMR. Also, highly concentrated R4 solutions (>4 mg ml −1 ) become cloudy above 15 °C, but re-clear upon cooling to 5 °C, suggesting reversible oligomerization, or aggregation, of R4 mediated by hydrophobic interactions (all biophysical experiments were thus conducted at 5 °C unless otherwise stated). R4 aggregation was increased at the high protein concentrations required for resonance assignment spectra, which precluded direct assignments; however, we obtained unequivocal assignments of 138 peaks to individual R4 residues by overlaying the R4 HSQC with the highly similar HSQC of an R4 derivative (R4 ΔH1 ). The correlation of these assignments with secondary structure likelihood (based on TALOS+) [21] revealed that the α-helices match those in the crystal ( Supplementary Fig. S6 ), indicating similar crystal and solution structures of R4. Next, we challenged 15 N-labelled R4 with equimolar amounts of CA (100 μM each), but this resulted in protein precipitation and >90% loss of the overall signal HSQC intensity relative to that of untreated R4. To avoid precipitation, we reduced the CA and R4 concentrations to 50 μM each, which resulted in an HSQC showing signs of exacerbated R4 aggregation because of CA (with signal intensities tending to be higher within the 8–8.6 p.p.m. range, but lower outside it; Fig. 3c ). We used right-angle light scattering to demonstrate directly that CA stimulates R4 aggregation ( Supplementary Fig. S7 ). The R4+CA spectrum also reveals a small subset of discrete peaks (including 9 that can be correlated confidently with the assigned HSQC; Supplementary Fig. S6 ) that exhibit a more pronounced exchange broadening upon CA exposure ( Fig. 3d , purple) compared with the majority of the peaks. Mapping these onto the R4 crystal structure ( Fig. 3e ) reveals an internal cluster underneath H1 ( Fig. 3d , black dots), possibly responding to CA binding to the surface above, and two CA responsive valines ( Fig. 3d , arrowheads) at the HD2-binding surface, which contribute to the 'acidic knob' crucial for the HD2 interaction [18] (whereby V167 directly contacts HD2; Fig. 3f ), perhaps explaining why CA disrupts ARD-HD2 binding. A third site is revealed at the C-terminus, which may be involved in oligomerization (see below, Supplementary Fig. S8 ). The structurally labile H1 is required for the CA response The above-described experiments did not allow us to probe the H1 residues (N141–A149) for their CA response, as these are intrinsically unstructured and missing in the assigned HSQC ( Supplementary Fig. S6 ). Recall that H1 adopts a helical structure if the ARD is complexed with BCL9 (ref. 18 ; Supplementary Fig. S3 ), and also with other ligands ( Supplementary Table S5 ) including E-cadherin [22] and α-catenin [23] , the latter being the only known ligand that interacts with H1 directly. Intriguingly, the aromatic ring of Y142 at the H1 N-terminus contributes to the hydrophobic core of a four-helix bundle between α- and β-catenin [23] , and it was proposed that the hydrophobic C-terminus of E-cadherin (which binds to the hydrophobic surface of the ARD N-terminus) could shield β-catenin from aggregation and proteasome-mediated destruction [22] . We thus conjectured that H1 might be responsible for the observed oligomerization of R4, and perhaps even contain the CA-binding site. To test this, we deleted amino acids N141–A149 from R4 (R4 ΔH1 ), which resulted in a much improved HSQC, stable over weeks (at 5–15 °C) and with relatively homogeneous peak intensities throughout ( Fig. 4a ), indicating that R4 ΔH1 is less prone to aggregation than R4. This allowed us to assign 138 backbone amide peaks to individual R4 ΔH1 residues ( Supplementary Fig. S6 ). As mentioned, the overlay of the R4 ΔH1 and R4 spectra exhibits a high similarity, indicating an overall similar structural fold. The projection of the chemical shift differences onto the R4 sequence and crystal structure reveals that the majority of the R4 residues affected by the presence of H1 cluster at the R4 N-terminus, immediately adjacent to H1 ( Supplementary Fig. S8 ). A second cluster is observed at the R4 C-terminus ( Supplementary Fig. S8 , asterisks), highlighting a surface-exposed hydrophobic patch that might be involved in oligomerization. 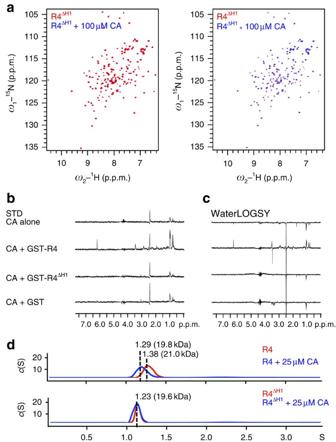Figure 4: The CA response of R4 depends on H1. (a) Overlay of HSQCs of15N-labelled R4ΔH1+CA (100 μM each; blue) onto R4ΔH1-CA (100 μM; red), and inverted spectral overlay (right-hand panel). (b,c) STD and WaterLOGSY spectra of 50 μM CA alone (reference), or +10 μM GST-tagged proteins, as indicated. (d) Sedimentation velocity AUC of His-R4 or His-R4ΔH1±CA (25 μM each), as indicated. Molecular masses were determined from corresponding sedimentation coefficient values (S), by modelling R4 and R4ΔH1as spherical proteins, using SedFit53. Figure 4: The CA response of R4 depends on H1. ( a ) Overlay of HSQCs of 15 N-labelled R4 ΔH1 +CA (100 μM each; blue) onto R4 ΔH1 -CA (100 μM; red), and inverted spectral overlay (right-hand panel). ( b , c ) STD and WaterLOGSY spectra of 50 μM CA alone (reference), or +10 μM GST-tagged proteins, as indicated. ( d ) Sedimentation velocity AUC of His-R4 or His-R4 ΔH1 ±CA (25 μM each), as indicated. Molecular masses were determined from corresponding sedimentation coefficient values (S), by modelling R4 and R4 ΔH1 as spherical proteins, using SedFit [53] . Full size image Importantly, the HSQC of R4 ΔH1 remains essentially unchanged upon stoichiometric addition of CA ( Fig. 4a; Supplementary Fig. S9 ). Likewise, there is virtually no CA response of R4 ΔH1 as judged by right-angle light scattering ( Supplementary Fig. S7 ). Consistent with this, ligand-observed binding assays (STD and WaterLOGSY) demonstrate that CA does not bind to GST-R4 ΔH1 ( Fig. 4b,c ). Thus, H1 contains, or contributes to, the primary CA-binding site within R4. This implies that the CA-induced line broadenings described above ( Fig. 3d ) largely reflect indirect consequences of CA's binding to H1—for example, increased R4 aggregation and/or conformational modulation. Close inspection of the R4/R4 ΔH1 HSQC overlay reveals a small number of major unassigned peaks that are R4 specific (that is, likely to originate from H1 residues), all poorly resolved and exhibiting random coil-like H N chemical shifts in the 7.9–8.6 p.p.m. range ( Supplementary Fig. S10 , boxed), consistent with unstructured polypeptide. A subset of these undergo CA-induced line broadening or slight chemical shift perturbations, and may thus reflect H1 residues within the primary CA-binding site. To obtain NMR-independent evidence that the CA response depends on H1, we conducted analytical ultracentrifugation (AUC). Velocity AUC reveals a sedimentation coefficient of 1.38 for R4, corresponding to an apparent molecular mass of ! kDa for a spherical globular protein (demonstrating that R4 is monomeric under these conditions). Stoichiometric addition of CA shifts this coefficient to 1.29, corresponding to an apparent reduction in molecular mass (19.8 kDa; Fig. 4d , top), consistent with a CA-induced shape change of R4 towards a less compact state (oligomerization is not apparent under these conditions). In contrast, R4 ΔH1 sediments with a coefficient of 1.23 (corresponding to an apparent molecular mass of 19.6 kDa), which remained unchanged upon addition of CA ( Fig. 4d , bottom), confirming that the CA response of R4 depends on H1. CA inhibits β-catenin-dependent transcription Having identified β-catenin as a direct CA target, we asked whether CA would affect its activity in cell-based assays. Toxicity assays showed that CA, 684 and 291 are well tolerated by cells, whereas CO and 986 compromised cell viability at high concentrations (≥40 μM), and totarol was highly toxic ( Supplementary Fig. S11 ). The latter two were not pursued as their substantial cell toxicity would complicate the interpretation of their effects on specific β-catenin-dependent readouts. We tested the non-toxic compounds for their ability to inhibit β-catenin activity, monitoring the transcript levels of the universally Wnt-inducible gene AXIN2 (ref. 24 ), and also of another Wnt target gene, B9L [14] , relative to an internal control ( TBP ). Treatment of HeLa cells with 20 mM LiCl (to block GSK3) increased the transcript levels of the Wnt target genes two to six times ( Fig. 5a ), which was unaffected by 291 or 684, possibly because these compounds are not taken up by the cells. In contrast, 25 μM CA reduced Wnt target gene transcripts to 40% ( AXIN2 ) and 60% ( B9L ) of mock-treated control cells, without affecting HPRT expression, whereas CO decreased expression of all three genes indiscriminately ( Fig. 5a ). Similar results were obtained with colorectal cancer cells (SW480 cells expressing mutant APC , and HCT116 cells expressing unphosphorylatable β-catenin): no effects of 291 and 684, selective attenuation of Wnt target genes by CA, and indiscriminate effects of CO ( Fig. 5b ; Supplementary Fig. S12 ). 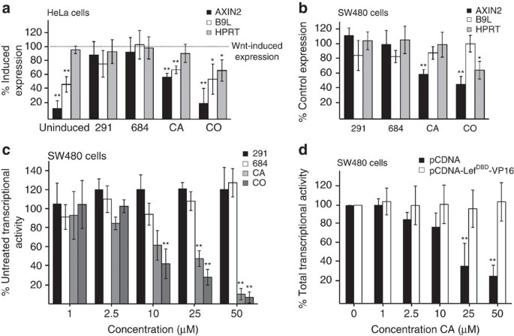Figure 5: CA inhibits β-catenin activity in human cells. (a,b) Real-time quantitative PCR analysis in (a) LiCl-stimulated HeLa or (b) SW480 cells, exposed to 25 μM compound for 6 h as indicated (explanations as inFig. 2). Percent reductions of transcript levels relative to (a) DMSO-treated LiCl-induced control or (b) DMSO-treated control values are shown at the *P<0.01 and **P<0.001 significance levels. (c,d) TOPFLASH assays in SW480 cells, transfected with (c) empty vector or (d) LEF-VP16 transactivator, on treatment with increasing concentrations of compound as indicated; reductions of relative luciferase values as percentage of DMSO-treated control values are shown; significance as inaandb. Error bars, standard deviations (n=4). Figure 5: CA inhibits β-catenin activity in human cells. ( a , b ) Real-time quantitative PCR analysis in ( a ) LiCl-stimulated HeLa or ( b ) SW480 cells, exposed to 25 μM compound for 6 h as indicated (explanations as in Fig. 2 ). Percent reductions of transcript levels relative to ( a ) DMSO-treated LiCl-induced control or ( b ) DMSO-treated control values are shown at the * P <0.01 and ** P <0.001 significance levels. ( c , d ) TOPFLASH assays in SW480 cells, transfected with ( c ) empty vector or ( d ) LEF-VP16 transactivator, on treatment with increasing concentrations of compound as indicated; reductions of relative luciferase values as percentage of DMSO-treated control values are shown; significance as in a and b . Error bars, standard deviations ( n =4). Full size image We also used the well-established TOPFLASH reporter assay [25] in SW480 cells, to test our compounds in this direct and highly specific assay for β-catenin-dependent transcription. Again, 291 and 684 showed no effect while both CA and CO consistently inhibited TOPFLASH to ~10% of the control ( Fig. 5c ), but CO also reduced the absolute renilla values (used as internal control) at ≥25 μM, confirming that this compound lacks specificity. Importantly, a VP16-LEF1 chimera whose transcriptional activity depends exclusively on the viral transactivation domain [26] was completely refractory to CA inhibition in this assay ( Fig. 5d ), demonstrating that the CA response of this transcriptional assay is conferred by β-catenin. CA targets activated β-catenin for proteasomal degradation Given that CA destabilizes R4 in vitro , we wondered whether it would also destabilize β-catenin in vivo , earmarking it for proteasomal degradation [27] . We thus monitored the levels of active β-catenin in CA-treated SW480 cells (which are high, because of their APC mutation) with an antibody specific for unphosphorylated β-catenin (called α-ABC [28] ). Strikingly, exposure of these cells to 25 μM CA reduces the α-ABC-reactive β-catenin pool relatively rapidly, and time dependently, to <30% of control levels ( Fig. 6a ; for a dose response, see Supplementary Fig. S13 ). By contrast, there is no significant reduction if the same lysates are probed with antibodies against phosphorylated β-catenin, total β-catenin (most of which, in epithelial cells, represents the E-cadherin-bound pool; see Discussion ), E-cadherin or α-catenin ( Fig. 6b ; Supplementary Fig. S13 ). Importantly, high levels of unphosphorylated β-catenin are restored in CA-treated cells if their proteasomes are inhibited by MG132 ( Fig. 6b ), lactacystin or epoxomycin ( Supplementary Fig. S14 ). By contrast, the levels of inhibitor of κB (IκB; whose proteasomal degradation is controlled by the same SCF β−TrCP ubiquitin ligase as β-catenin [29] ) are barely affected by CA ( Fig. 6b ), even after 20 h of treatment. Thus, CA promotes selectively the proteasomal degradation of oncogenic β-catenin in colorectal cancer cells. In support of this, the half-life of unphosphorylated β-catenin is reduced significantly by CA, from ~7 h in untreated cells to 3–4 h in CA-treated cells ( Supplementary Fig. S15 ). 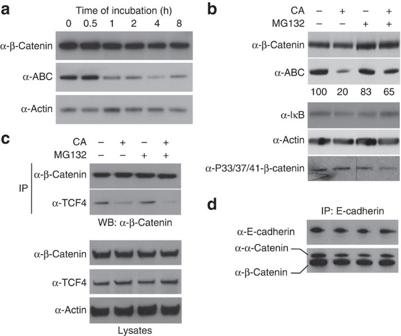Figure 6: CA destabilizes oncogenic β-catenin in colon cancer cells. (a,b) Western blots of SW480 cell lysates, (a) treated with 25 μM CA for periods indicated above panels or (b) simultaneously treated with 25 μM CA±10 μM MG132 for 4 h, probed with antibodies as indicated (see alsoSupplementary Fig. S8); percent reductions of unphosphorylated β-catenin (measured by densitometry of α-ABC bands) are given underneath panel. (c) Western blots (WB) of lysates from mock- or CA-treated SW480 cells (for 6 h) ±10 μM MG132 (for the last 4 h), after immunoprecipitation (IP) and probing (WB) with antibodies as indicated (total lysates, underneath). (d) Western blots of the same SW480 cell lysates shown inb, after IP with E-cadherin antibody, probed with antibodies as indicated on the left. Figure 6: CA destabilizes oncogenic β-catenin in colon cancer cells. ( a , b ) Western blots of SW480 cell lysates, ( a ) treated with 25 μM CA for periods indicated above panels or ( b ) simultaneously treated with 25 μM CA±10 μM MG132 for 4 h, probed with antibodies as indicated (see also Supplementary Fig. S8 ); percent reductions of unphosphorylated β-catenin (measured by densitometry of α-ABC bands) are given underneath panel. ( c ) Western blots (WB) of lysates from mock- or CA-treated SW480 cells (for 6 h) ±10 μM MG132 (for the last 4 h), after immunoprecipitation (IP) and probing (WB) with antibodies as indicated (total lysates, underneath). ( d ) Western blots of the same SW480 cell lysates shown in b , after IP with E-cadherin antibody, probed with antibodies as indicated on the left. Full size image As an independent measure of the transcriptionally active β-catenin, we quantified the levels of TCF4-associated β-catenin in CA-treated SW480 cells by TCF4 co-immunoprecipitation. Once again, the total β-catenin levels are little affected by CA, but the levels of TCF4-associated β-catenin are substantially reduced compared with their controls ( Fig. 6c ). In contrast, the E-cadherin-associated β-catenin and α-catenin are barely affected by CA ( Fig. 6d ). We note that MG132 does not restore the association of β-catenin with TCF4 in CA-treated cells ( Fig. 6c ), possibly because the CA-induced conformer of β-catenin that accumulates during proteasome inhibition may not be fully folded and, thus, unable to gain access to the nucleus and/or chromatin-bound TCF4. Next, we asked whether H1 is responsible for the CA-induced degradation of activated β-catenin. LiCl treatment of HEK 293 cells transfected with FLAG-β-catenin causes an increase of unphosphorylated FLAG-β-catenin, which is reduced in a dose-dependent manner by CA ( Fig. 7a ). Importantly, FLAG-β-catenin with an internal deletion of H1 (FLAG-β-catenin ΔH1 ) does not respond to CA, and its levels are maintained up to 25 μM CA ( Fig. 7a ). This is fully consistent with our biophysical evidence that the CA response of R4 depends on H1. 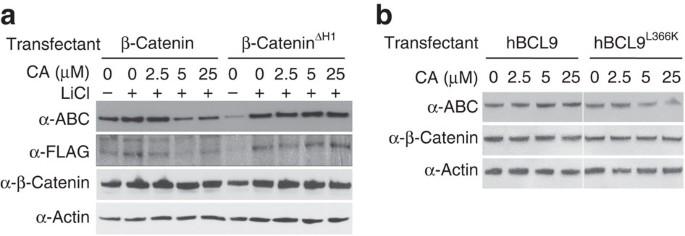Figure 7: CA-induced destabilization of active β-catenin depends on H1. Western blots of lysates from HEK 293 cells, transfected with (a) FLAG-β-catenin or FLAG-β-cateninΔH1, or (b) FLAG-BCL9 or FLAG-BCL9L366K, mock-treated or after simultaneous exposure to 20 mM LiCl and CA (0–25 μM) for 6 h, probed with antibodies as indicated. Figure 7: CA-induced destabilization of active β-catenin depends on H1. Western blots of lysates from HEK 293 cells, transfected with ( a ) FLAG-β-catenin or FLAG-β-catenin ΔH1 , or ( b ) FLAG-BCL9 or FLAG-BCL9 L366K , mock-treated or after simultaneous exposure to 20 mM LiCl and CA (0–25 μM) for 6 h, probed with antibodies as indicated. Full size image Interestingly, overexpressed BCL9 protects β-catenin slightly from CA destabilization in SW480 cells, whereas the L366K mutant provides no protection ( Fig. 7b ). Protection is also afforded by an overexpressed C-terminal truncation of BCL9, but not by its L366K mutant version ( Supplementary Fig. S16 ). Thus, the binding of BCL9 to the ARD N-terminus can protect β-catenin against CA-induced destabilization. We described a 'plus–minus' screen that led to the discovery of the rosemary compound CA, which inhibits the binding of β-catenin to BCL9 in vitro , and which reduces the levels of oncogenic β-catenin in vivo , thus attenuating its transcriptional outputs. Our counter-screen allowed us to distinguish general chaotropic agents from compounds that specifically affect the HD2-ARD but not the nTCF-ARD interaction, which proved invaluable to discard unspecific hitters, which were prevalent in all three screens. The only three hits that survived the counter-screen came from the Phytopure library, suggesting that natural product libraries provide a useful source of compounds for disrupting protein–protein interactions. These Phytopure hits led us to identify CA, the major phenolic diterpene in rosemary leaf extracts (constituting ~4% of their dry weight; see also ref. 30 ). Together with CO, CA is responsible for the antioxidant activity of rosemary extracts [31] , which apparently accounts for their potent anti-inflammatory and anti-tumourigenic effects [32] , and also for the neuroprotective effects of CA in cell culture and mouse brains [33] . Our NMR studies identified β-catenin as a direct molecular target of CA. Three lines of evidence argue that the observed in vitro effects of CA on R4 could explain its in vivo effects on β-catenin. First, the CA-induced reduction of the cellular β-catenin levels is relatively rapid and dose dependent, consistent with a direct response. Second, the IC 50 s of the cellular responses of CA overlap its K i for interfering with HD2-ARD binding, its K d for binding to R4, and they are within the range of CA concentrations that promote in vitro aggregation of R4. Third, and most important, deletion of H1 eliminates the CA response of R4 in vitro , and that of β-catenin in vivo . This excellent correlation between in vitro and in vivo effects of CA is consistent with the latter reflecting the former, which we shall take to be the case below—bearing in mind that CA could have additional cellular targets that might affect β-catenin stability and outputs. Our biophysical data suggest that H1 contains, or contributes to, the CA-binding site of R4, and that CA acts through H1 to exacerbate an intrinsic tendency of the ARD N-terminus to aggregate. Given that H1 is intrinsically unstructured [19] , and our evidence from AUC for a CA-induced R4 shape change, it is conceivable that CA, on binding to the ARD N-terminus, induces a conformational change of H1, which favours aggregation. Indeed, CA may fix H1 in a conformation that is incompatible with its folding into the helical structure necessary for accommodating HD2 (ref. 18 ; Supplementary Fig. S3 ), which would explain why CA interferes with HD2-ARD binding. Recall also that CA does not interfere with ARD binding to nTCF (predominantly involving residues downstream of R4 (ref. 34 )), further supporting the notion that the CA-induced perturbations are limited to the ARD N-terminus. In the light of our in vitro observations, we propose that the metastable H1 also predisposes β-catenin to low-grade aggregation in vivo , and that this is exacerbated by CA, which could earmark β-catenin for proteasomal degradation [27] , [35] ( Fig. 8 ). This model could explain why the phosphorylated pool of β-catenin (which in epithelial cells includes junctional β-catenin) [36] , [37] is refractory to CA: this β-catenin pool is complexed with E-cadherin, a high-affinity ligand (with a K d of ~100 times below the K i for CA inhibition) [38] that confers a helical structure on H1, and protects it from CA inhibition. Note also that β-catenin associates with E-cadherin co-translationally [39] , [40] , which would safeguard it against H1-mediated CA effects from its de novo synthesis. 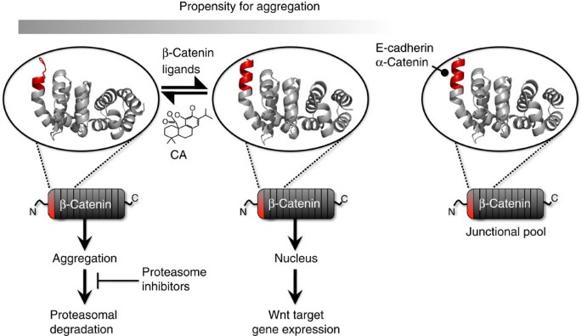Figure 8: Model of CA-induced proteasomal degradation of β-catenin. Unphosphorylated β-catenin (signalling pool, accumulating during Wnt signalling; or oncogenic pool, accumulating in colorectal cancer cells due toAPCorβ-cateninmutations) is inherently prone to low-level aggregation due to the structurally labile H1 (red, at the ARD N-terminus). H1 adopts a helical conformation (red ribbon) upon binding to ligands (for example, BCL9), which is reversed towards a less ordered state by CA; this exacerbates the intrinsic tendency of β-catenin to aggregate, earmarking it for proteasomal degradation. Phosphorylated β-catenin is targeted for proteasomal degradation upon binding to Axin (not shown), or stabilized by binding to E-cadherin or α-catenin (destined for the junctional pool), which ensure a helical conformation of H1. Figure 8: Model of CA-induced proteasomal degradation of β-catenin. Unphosphorylated β-catenin (signalling pool, accumulating during Wnt signalling; or oncogenic pool, accumulating in colorectal cancer cells due to APC or β-catenin mutations) is inherently prone to low-level aggregation due to the structurally labile H1 (red, at the ARD N-terminus). H1 adopts a helical conformation (red ribbon) upon binding to ligands (for example, BCL9), which is reversed towards a less ordered state by CA; this exacerbates the intrinsic tendency of β-catenin to aggregate, earmarking it for proteasomal degradation. Phosphorylated β-catenin is targeted for proteasomal degradation upon binding to Axin (not shown), or stabilized by binding to E-cadherin or α-catenin (destined for the junctional pool), which ensure a helical conformation of H1. Full size image According to our model, H1 constitutes an Achilles' Heel of β-catenin, which, in the absence of ligands that stabilize its structure in a helical conformation [18] , [22] , [23] , earmarks it for proteasomal turnover in cells by promoting localized structural perturbations that favour low-grade aggregation. Notably, an unstructured H1 is also found in β-catenin of other species ( Supplementary Table S5 ), so this Achilles' Heel appears to be conserved. Perhaps, this feature serves as a last-resort tagging mechanism to prevent fortuitous activation of β-catenin, should it fail to bind to its negative regulators. Indeed, H1-dependent proteasomal degradation of β-catenin could be particularly important when its negative regulators are rate limiting, or absent—for example, in colorectal cancer cells with dysfunctional APC, and low E-cadherin levels [37] . This may render oncogenic β-catenin particularly vulnerable and prone to degradation, a property shared by other oncogenes whose stability is reliant on chaperones such as HSP90 (refs 41 , 42 ). BCL9 family proteins shuttle in and out of the nucleus [43] , and could thus convey β-catenin from the cytoplasm to chromatin-bound Pygo at TCF-target genes [44] . Interestingly, excess BCL9 protects unphosphorylated β-catenin against CA-induced degradation, possibly by promoting a helical structure of H1. BCL9 may thus have a chaperone-like ('shepherding') role in protecting oncogenic β-catenin against H1-dependent degradation. We note that BCL9 is a lower-affinity ligand of β-catenin compared with E-cadherin, and may thus need to be present at high levels to afford protection. BCL9 proteins are overexpressed in colorectal cancer cells and carcinomas [12] , [13] , [14] , [15] and may thus be effective in safeguarding oncogenic β-catenin against H1-dependent degradation. β-Catenin is an unattractive drug target, because of its extensive interaction surfaces with TCF and negative regulators [4] . Our discoveries of an Achilles' Heel at its N-terminus, and of a H1-dependent compound destabilizing oncogenic β-catenin, open up avenues for new screen designs, such as inhibiting R4's interaction with other 'shepherding' ligands of β-catenin—similar to a promising strategy aimed at inhibiting oncogene interactions with their stabilizing HSP90 chaperone [42] . Indeed, as exemplified by a recent study with c-Myc [45] , the targeting of intrinsically disordered stretches of proteins such as H1 is an emerging strategy in drug discovery [46] . Chemicals and antibodies Chemicals: dimethyl sulphoxide (DMSO), totarol, CO, CA (Sigma); glutathione-coated 96- and 384-well microtiter plates (Pierce); 15 N-ammonium chloride, 13 C-glucose (Isotec). Antibodies: α-β-catenin (BD Transduction Laboratories); α-ABC, α-α-catenin (Upstate); α-phospho-β-catenin (Ser33/37/Thr41; Cell Signalling); α-IκB (Santa Cruz); α-actin (Abcam); α-E-cadherin, α-FLAG (Sigma). Plasmids and protein expression Plasmids: FLAG-β-catenin (from H. Clevers); FLAG-BCL9 and mutants [14] ; and GST-ARD [19] . For FLAG-β-catenin ΔH1 , amino acids 141–149 were excised by quick-change mutagenesis (Stratagene). nTCF (1–53 from hTCF4) and HD2 (343–396 from hBCL9) were cloned into pET30a, and mutations were introduced into pET30a-HD2 by quick-change mutagenesis. R4 (141–305) and R4 ΔH1 (149–305) were cloned into pETM11 or pGEX-4T1. Protein was expressed at 18 °C in Escherichia coli BL21, induced by 1 mM isopropyl β- D -1-thiogalactopyranoside at 1.0 OD for 16 h, and purified with glutathione Sepharose 2B (AP Biotech) or Ni-NTA Agarose (Qiagen), followed by Superdex-75 size exclusion chromatography, with phosphate-buffered saline (PBS, pH 7.4) as running buffer for GST-ARD, GST and His-nTCF, or with PBS (pH 6.8) plus 100 mM NaNO 3 for His-R4 and His-HD2. For NMR, untagged versions of R4 and R4 ΔH1 were generated by thrombin digestion, followed by size exclusion chromatography. His-HD2 was cleaved with enterokinase, and tag and undigested protein were cleared from tag-free HD2 by negative absorption with Ni-NTA Agarose. For HSQC, 15 N-, 2 H/ 13 C- and 2 H/ 13 C/ 15 N-labelled domains were produced from bacteria grown in minimal media containing 15 N-ammonium chloride or, additionally, 13 C 6 -glucose and/or in D 2 O instead of water. Compound libraries and screening For the LOPAC (Sigma) and Phytopure (Phytoquest Ltd) screens, 10 μg of GST-ARD (or GST as control) in PBS containing 1% bovine serum albumin and 0.1%. Tween-80 (blocking buffer) was adsorbed to wells in 96-well glutathion-coated microplates (Pierce; we could not detect binding after direct coating of ARD or GST-ARD onto plastic, nor after immobilization of GST-HD2 or His-HD2 on microplates); volumes were kept at 50 μl. Wells were incubated with His-HD2 or His-nTCF (10 μM) in blocking buffer and, subsequently, with 20 μM of compounds diluted in PBS; remaining His-HD2 or His-nTCF was detected by adsorption of horse radish peroxidase-coupled α-His antibody followed by development with 100 μl O -phenylenediamine reagent (Sigma) and spectrophotometric quantification. A hit was defined as a signal >3 standard deviations below that of mock-treated wells containing GST-ARD and His-HD2. Hits were defined as confirmed if the signal in the counter-screen was within 0.5 standard deviations of mock-treated wells. The MRCT library and its screen are described in the Supplementary Table S1 and Figure S2 . Cell-based assays SW480, HCT116, HeLa and HEK 293 cells (obtained from the European Collection of Cell Cultures) were grown and transfected, and reporter assays and real-time quantitative PCR were done as described [14] . Cytotoxicity assays are described in the Supplementary Figure S11 . NMR spectroscopy All NMR experiments were recorded using Bruker spectrometers equipped with 5 mm cryogenic inverse triple resonance probes, at a sample temperature of 5 °C unless stated otherwise. 1 H, 15 N-fast-HSQC spectra [47] were acquired on 700 or 800 MHz spectrometers. Raw data (1,024 points in t 2 , 96 complex points in t 1 extended to 128 by forward linear prediction) were processed with 85° shifted square-sine-bell functions in both directions before Fourier transformation. The digital resolution of processed data was 5.4 Hz per point in f 2 ( 1 H) and 2.7 Hz per point in f 1 . Effective molecular weight estimates were obtained from two one-dimensional spin-echo spectra, used to estimate average amide- 1 H T 2 for 1 H frequencies >8.6 p.p.m., and to infer an approximate rotational correlation time and, hence, molecular weight, as described [20] . Samples were maintained at 5 °C in PBS (pH 6.8) containing 100 mM NaNO 3 , 5% (v/v) D 2 O. Chemical shifts were internally referenced using the frequency of H 2 O resonance as secondary reference. Resonance assignments of R4 ΔH1 and HD2 are described in the Supplementary Figures S5 and S6 . Ligand-observed NMR experiments were carried out with excitation sculpting water signal suppression at 500 MHz. WaterLOGSY spectra [48] were acquired with 4,096 points, 6 kHz spectral width, 25 ms 3-Gaussian 180° water selection pulse, 0.9 s NOE mixing time, and 2.5 s relaxation delay, 2,000 scans, and a T 1 ρ filter (50 ms square pulse with 2.2 kHz B 1 field) to suppress signals from protein. STD spectra [49] were acquired using a pseudo-2D pulse sequence (unmodified Bruker pulse program stddiffesgp.3), 16k or 8k points, 8 kHz spectral width, 512 scans, interleaving on-resonance (−0.2 p.p.m.) or off-resonance (25.2 p.p.m.) pre-saturation (repeating 50 ms 1% truncated Gaussian pulses with 105 Hz B 1 field) throughout the 7.0 s recycle delay, and a 15 ms T 1 ρ trim pulse (square pulse, 5.8 kHz B 1 ). Titrations based on STD were done as described [50] ; average spectral intensities at varying protein concentration were fitted to single-site-binding using Prism software. Addition of CA (in DMSO), or DMSO only, to all NMR samples was standardized to 4.5% total sample volume. All NMR spectra were processed with TopSpin version 2 (Bruker). Multidimensional spectra were analysed using Sparky 3.110 (T. D. Goddard & D. G. Kneller, University of California, San Francisco). X-ray crystallography Laboratory of Molecular Biology (LMB) crystallization screens were carried out in 96-well sitting-drop format (100 nl drops) [51] . Crystals were grown at 19 °C by the vapour diffusion method, and emerged after a week under multiple conditions. Crystals for data collection were from the following conditions: 0.98 M sodium acetate trihydrate, 30% glycerol, 0.07 M sodium cacodylate (pH 6.5), 30% (w/v) galactose (R4); 0.12 M ethylene glycol, 1 M MES and 1 M imidazole (pH 6.5), 10% PEG 4K, 20% glycerol (R4-HD2). Crystals were flash-cooled in liquid nitrogen, and diffraction data were collected at SLS X06SA and ESRF ID14-2 for the R4 and R4-HD2 structures, respectively, at wavelength 0.93 Å. Structures were solved by molecular replacement (with phaser [52] based on the ARD-HD2–nTCF complex [18] ), processed and refined as described in the Supplementary Table S4 and Figure S3 . Analytical ultracentrifugation AUC was performed with a Beckman Coulter Optima XL-I ultracentrifuge (Beckman Coulter) and data collected with Rayleigh interference optics. Samples in PBS (pH 6.8) containing 100 mM NaNO 3 were equilibrated in the cell at 5 °C for >3 h before the run, during which interference data were collected. Accession codes: Coordinates and structure factors have been deposited with the Protein Data Bank under accession codes 3SLA and 3SL9 . How to cite this article: de la Roche, M. et al . An intrinsically labile α-helix abutting the BCL9-binding site of β-catenin is required for its inhibition by carnosic acid. Nat. Commun. 3:680 doi: 10.1038/ncomms1680 (2012).